Metabolic efficiency underpins performance trade-offs in growth ofArabidopsis thaliana Growth often involves a trade-off between the performance of contending tasks; metabolic plasticity can play an important role. Here we grow 97 Arabidopsis thaliana accessions in three conditions with a differing supply of carbon and nitrogen and identify a trade-off between two tasks required for rosette growth: increasing the physical size and increasing the protein concentration. We employ the Pareto performance frontier concept to rank accessions based on their multitask performance; only a few accessions achieve a good trade-off under all three growth conditions. We determine metabolic efficiency in each accession and condition by using metabolite levels and activities of enzymes involved in growth and protein synthesis. We demonstrate that accessions with high metabolic efficiency lie closer to the performance frontier and show increased metabolic plasticity. We illustrate how public domain data can be used to search for additional contending tasks, which may underlie the sub-optimality in some accessions. Living organisms perform many different and sometimes contending tasks, leading to trade-offs in which optimal performance of one task comes at the cost of a sub-optimal performance of another task. Trade-offs are influenced by the environment and their resolution depends on metabolic resources and plasticity [1] , [2] . One important environmental variable affecting plant growth is resource availability [3] , [4] , [5] , [6] . We first ask whether there is a trade-off between two tasks during vegetative growth of Arabidopsis thaliana : the maximization of physical size and the maximization of protein concentration. We then apply two methods to rank accessions: the first based solely on the performance of tasks, and the second based on the efficiency with which metabolic resources are deployed to perform tasks. In addition, we investigate whether the trade-off and the ranking of accessions are affected by the availability of carbon (C) and nitrogen (N) and the way in which it shapes the accession-specific metabolic profiles. Plants use light energy to transform CO 2 and inorganic nutrients into a plethora of metabolic precursors that are used to drive growth. As plants are sessile, resource acquisition is constrained by their physical size. In land plants, the majority of a mature cell is occupied by the vacuole, allowing the generation of a much larger physical size per unit protein than is usually obtained by microbes or animals [7] . For simplification, we do not consider the impact of shape and phenology on the relation between physical size and resource acquisition. On the other hand, proteins are required to catalyse the transformation of resources into biomass. In particular, the majority of the protein in a plant leaf is involved in photosynthesis [8] , [9] , [10] . We hypothesize that there is a trade-off between physical size and protein concentration. While production of leaves with a higher protein concentration will allow higher rates of photosynthesis and metabolism per unit biomass, it also increases the costs of growth and decreases physical size, resulting in the occupation of less space and the acquisition of smaller amounts of resources. In particular, a decrease in rosette area will decrease how much light is intercepted [7] , [11] , [12] . Plant size and protein concentration will additionally strongly depend on growth conditions, especially those affecting resource supply and allocation, such as daily irradiance and nitrogen availability [13] , [14] . Trade-offs between tasks are not measured directly but are rather inferred from measurements of the corresponding phenotypic traits. To study the effect of resource acquisition and allocation on trade-offs, the contending traits are measured along two orthogonal axes. One axis is given by a collection of genotypes, for example, accessions or species, and the other by differing environments. Inference of trade-offs from the resulting large multidimensional data set of trait scores is typically based on correlation-driven methods. However, while a negative correlation between two traits may be indicative of trade-off [15] , [16] , it does not reveal what underlies the trade-off. Furthermore, correlation-driven methods do not allow the quantification and comparison of trade-offs in individual genotypes and under different conditions. This led us to ask whether more information can be extracted using the Pareto performance and efficiency frontiers [17] , [18] , [19] , [20] , [21] originating in engineering and the social sciences. While there can be many feasible strategies to allocate resources to contending tasks, only a few of them result in an optimal trade-off [21] , [22] , [23] . A strategy, corresponding to a genotype [24] in a given condition, provides an optimal trade-off when a further increase in the performance of one task is not possible without decreasing the performance of other tasks. 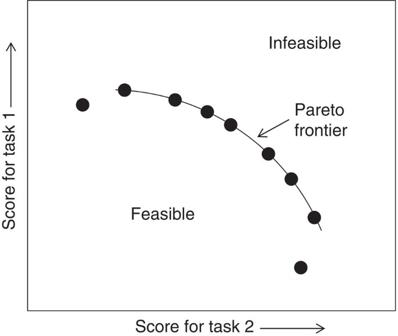Figure 1: Pareto performance concept. Schematic illustration of Pareto performance. Two contending tasks are studied in one condition. The performance of genotypes is scored with respect to the two tasks and is depicted by the two axes. Each genotype is represented as a point in the resulting 2D space. The genotypes with an optimal trade-off between the two tasks form the Pareto performance frontier. The frontier arises due to systemic constraints affecting the performance, and separates the feasible from the infeasible region. Figure 1 schematically illustrates a simple example in which two contending tasks are studied in one condition. Figure 1: Pareto performance concept. Schematic illustration of Pareto performance. Two contending tasks are studied in one condition. The performance of genotypes is scored with respect to the two tasks and is depicted by the two axes. Each genotype is represented as a point in the resulting 2D space. The genotypes with an optimal trade-off between the two tasks form the Pareto performance frontier. The frontier arises due to systemic constraints affecting the performance, and separates the feasible from the infeasible region. Full size image Four recent studies have illustrated the potential of the Pareto performance frontier to describe trade-offs at the phenotypic level: Shoval et al . [16] showed that trade-offs between tasks lead to Pareto fronts in the shape of simple polygons, for example, lines, triangles or tetrahedrons, in trait space. The vertices of the resulting polygons may be regarded as specialists for a single task, represented by a linear combination of traits. Sheftel et al . [25] extended this to show that slightly curved edges may arise under a wider range of assumptions. Szekely et al . [26] calculate the Pareto front of biological homeostasis circuits in the space of employed parameters. Moreover, Schuetz et al . [27] used a metabolic model to provide flux estimates [28] , and proposed that Escherichia coli has evolved towards optimal flux distributions in one condition while minimizing the changes required between conditions. The performance frontier provides a concise description of trade-offs, but does not explain why it adopts a given location, or why a particular genotype is located at or below the frontier ( Fig. 1 ). The location of a genotype is presumably constrained by the underlying factors that determine the trade-off between tasks. These factors can be analysed using the concept of relative Pareto efficiency [29] , [30] , which allows the comparison of different strategies for allocating finite amounts of resources between tasks. A resource allocation strategy is termed efficient if no other allocation strategy exists that is able to improve the performance of one task without decreasing the performance of other tasks or utilizing more of any individual resource [30] . Here we first illustrate how the performance frontier can be used to analyse and reduce a large multidimensional data set describing the trade-off between fresh weight and protein concentrations in A. thaliana natural accessions growing in three conditions. We regard metabolism as a production line with two outputs: protein and fresh weight, and use the metabolite and enzyme activity profiles to describe the structure and resource state of this production line. By using the Pareto efficiency concept, we ask whether the structure of this production line influences the trade-off between size and protein concentration in different accessions and conditions. The results reveal that while some accessions lie close to the performance frontier and are metabolically efficient, others show sub-optimality. As the findings of such analyses are contingent on the tasks, accessions and conditions used in the study, sub-optimality may indicate that the considered tasks are in trade-off with other tasks, examined by mining public domain data sources. Trade-off between fresh weight and protein concentration As a first step, we investigated whether there is a trade-off between production of rosette fresh weight and protein concentration in a panel of Arabidopsis accessions ( Supplementary Table 1 ). We rely on fresh weight, as it is the best indicator of plant size and is the key parameter in many allometric relationships [31] , [32] . Our analysis uses ex situ data collected on these two phenotypic traits and metabolic phenotypes in the rosette of the Arabidopsis accessions in three contrasting but not overly stressful growth conditions. The panel contained 97 accessions selected to show substantial genetic and geographical variation ( Supplementary Table 1 , Supplementary Fig. 1 ) [33] , [34] . The majority of the accessions come from Eurasia, together with some accessions from North America and Africa and derive from a range of growth habitats [35] , [36] . They were grown in a 8 h light/16 h dark photoperiod and high N supply in which growth was limited by C (LiC) [37] and in a 12 h light/12 h dark photoperiod at two levels of N fertilization, one allowing close to maximal growth (OpN) and another in which N limited the growth (LiN) [38] . The levels of 48 metabolites and the activities of eight enzymes in central metabolism were profiled to provide a metabolic phenotype in each growth condition ( Supplementary Methods ). When an increase in performance of one task results in a decrease in performance of another task, the corresponding traits will show a negative correlation. In our set of 97 accessions, the correlation between fresh weight and protein concentration was negative in all conditions: −0.30 ( P value=0.0032, t -distribution) for OpN, −0.40 ( P value=0.0877, t -distribution) for LiC and −0.17 ( P value=0.0001, t -distribution) for LiN (see Supplementary Fig. 2A–C , respectively). The negative relationship was strongest in LiC, and smaller and not significant in LiN, indicating that extent of the trade-off may be condition-dependent. A similar negative relationship was recently shown between N percentage, as a proxy of protein concentration, and the dry to fresh mass ratio in 122 vascular plant species [39] as well as between N content and leaf weight in barley [40] , demonstrating the generality of the trade-off between size and protein concentration within and across species, as well as its importance in an ecological context and in crop plants. Accession fresh weight between conditions correlated most strongly for the OpN/LiC comparison (0.47, P value=0, t -distribution), followed by LiC/LiN (0.31, P value=0.0017, t -distribution), and LiN/OpN (0.29, P value=0.0046, t -distribution) ( Supplementary Fig. 3A–C , respectively). The same order was obtained when protein concentration was used (0.34 ( P value=0.0006, t -distribution), 0.32 ( P value=0.0016, t -distribution) and 0.16 ( P value 0.1253, t -distribution) for OpN/LiC, LiC/LiN, and LiN/OpN, respectively) ( Supplementary Fig. 3D–F , respectively). These values indicated that the rankings of accessions based on a single task do not change dramatically between the three growth conditions, and point to a fairly robust trade-off situation in growth-related tasks. Average performance frontier While correlation analysis indicates that there may be a trade-off between two tasks, it does not provide accession-specific information about the performance of contending tasks and how this is affected by the growth condition. To provide this information, we investigated the trade-off between fresh weight and protein concentration with the help of the Pareto performance frontier. To obtain the performance frontier for a given condition, the accession with the highest performance for a given task is represented by a value of one, and all other accessions as a fraction of this value. When two (as in our case) or more tasks are considered, each accession is represented as a point in a two- or multi-dimensional space, respectively. The coordinates of the corresponding point are given by the normalized performance scores. The performance frontier for an investigated condition can be approximated by the bounding segments or, if there are more than two tasks, a surface from the convex hull connecting the best performers for each task. The resulting plots for each growth condition are provided in the Supplementary Information ( Supplementary Fig. 4A–C ). To obtain an average performance frontier, which summarizes the accession-specific trade-off between fresh weight and protein concentration in three contrasting environments, the following procedure was used (illustrated for Je-54 on Fig. 2 ). The scores for the performance of an accession with respect to its fresh weight and protein concentration in three conditions build a triangle for each accession. The centroid of the triangle corresponds to the average relative performance of each accession with respect to the two tasks. The extent to which performance was conserved between the three conditions is visualized by the size of the point, which is proportional to the area of the corresponding triangle; a small point denotes a conserved performance in the three conditions. The three lines arising from the centroid are directed towards the vertices of the triangle. 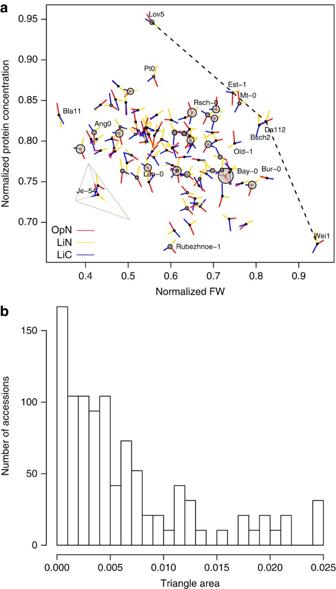Figure 2: Pareto performance frontier for the 97 considered Arabidopsis accessions. (a) The condition-specific normalized fresh weight (FW) and protein concentration provide the coordinates for the vertices of an accession-specific triangle, for example, forJe-54. The larger spread of FW in comparison to protein concentration is due to its nonlinear relationship to the relative growth rate. The average performance with respect to the two tasks across all three conditions is provided by the centroid of the triangle. The centroid is used as a representative of an accession, and the size of the associated point is proportional to the size of the respective triangle. The colour coding of the three lines incident on each centroid denotes the conditions, red for OpN, yellow for LiN and blue for LiC. The lines are directed towards the vertices of the corresponding triangle. For clarity, the vertices of the triangles are omitted from the plot. The dashed line approximates the Pareto performance frontier. (b) The histogram of accession-specific triangle areas for the three considered conditions suggests the presence of three groups of accessions: those performing similarly under all conditions (small triangle area), those differing in one condition (average triangle area) and those divergent in the three conditions (large triangle area). This procedure was repeated for all 97 accessions ( Supplementary Table 2 ). Figure 2: Pareto performance frontier for the 97 considered Arabidopsis accessions. ( a ) The condition-specific normalized fresh weight (FW) and protein concentration provide the coordinates for the vertices of an accession-specific triangle, for example, for Je-54 . The larger spread of FW in comparison to protein concentration is due to its nonlinear relationship to the relative growth rate. The average performance with respect to the two tasks across all three conditions is provided by the centroid of the triangle. The centroid is used as a representative of an accession, and the size of the associated point is proportional to the size of the respective triangle. The colour coding of the three lines incident on each centroid denotes the conditions, red for OpN, yellow for LiN and blue for LiC. The lines are directed towards the vertices of the corresponding triangle. For clarity, the vertices of the triangles are omitted from the plot. The dashed line approximates the Pareto performance frontier. ( b ) The histogram of accession-specific triangle areas for the three considered conditions suggests the presence of three groups of accessions: those performing similarly under all conditions (small triangle area), those differing in one condition (average triangle area) and those divergent in the three conditions (large triangle area). Full size image The visualization in Fig. 2 is more informative than a correlation-based analysis because it characterizes performance for multiple tasks and conditions in an accession-specific manner. Some accessions are better at accumulating protein, for example, Lov5 and Pt0 , as shown in the upper part of Fig. 2 , while others are better performers with respect to fresh weight, for example, Wei1 , Da112 , Bsch2 and Bur-0 , shown in the right part of Fig. 2 . From the distribution of areas of the triangles, shown in the inlay in Fig. 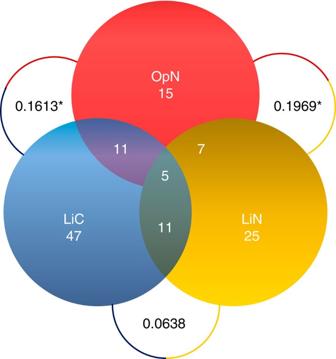Figure 3: Venn diagram of the number of efficient accessions under the three conditions. The number of efficient accessions based on the results from PCA–DEA with 70% of variance explained for the two outputs, fresh weight (FW) and protein concentration under OpN (red), LiN (yellow) and LiC (blue) conditions as well as shared efficient accessions between different conditions is presented in white. The Kendall tau correlation coefficient is presented in black. Significant Kendall tau correlation (Pvalue <0.05,zA-statistic) is marked with a star. 2 , we classified the accessions into three groups, supported by robust statistics ( Supplementary Table 3 ); the first group includes those performing similarly under all three conditions, for example, Bla11 , Da112 and Bur-0 , the second, those with similar performance under two conditions, for example, Bsch2 , Lan-0 and Pt0 , and third includes those with quite divergent relative performance in all conditions, for example, Bay-0 , Rubenzhnoe-1 , Mt-0 and Lov5 ( Supplementary Tables 3, 4 ). This classification is difficult to obtain by separate consideration of the three condition-specific performance frontiers ( Supplementary Fig. 4A–C ). The dashed lines in Fig. 2 connects the best average performer for fresh weight with the best average performer for protein concentration across all three conditions, using the bounding segments from the convex hull. These lines approximate to the average performance frontier of the three conditions. The distribution of accessions around this performance frontier was extremely unbalanced. Six accessions were close to or directly on the performance frontier, namely Wei1 , Bsch2 , Da112 , Mt-0 , Est-1 and Lov5 . To analyse the relationship between the distance from the average performance frontier and the trade-off between fresh weight and protein concentration, we calculated the correlation between fresh weight and protein concentration for groups of accessions, starting with the 10 closest to the frontier, and progressively increasing the set until it included all 97 accessions ( Supplementary Fig. 5 ). The negative correlation between fresh weight and protein was strongest for accessions closer to the average performance frontier, and became progressively weaker as more accessions were included. Figure 2 reveals that accessions lying well below the performance frontier fall into two groups; one shows a trend for a decreased fresh weight while retaining a relatively high protein concentration (an extreme representative of this group is Bla11 ), while the other group exhibits a trend for a decreased protein concentration while retaining a relatively high fresh weight (an extreme representative of this group is Rubezhnoe-1 ). Thus, this two-dimensional (2D) visualization of the average performance frontier provides insights into performance of two tasks across multiple conditions. However, in any given study, the location of the performance frontier is contingent on the investigated tasks, accessions and growth conditions, and that in particular the occurrence of additional tasks that are not considered in the analysis can lead to apparent sub-optimality. The occurrence of many accessions well below the performance frontier indicates that there may be more than the two investigated tasks in trade-off. To investigate this possibility, we also employed the approach of Shoval et al . [16] , which uses the criterion of triangularity with the data on fresh weight and protein concentration in each individual growth condition and their combination. This criterion was not significant at level α =0.01 (permutation test with 10,000 repetitions) ( Supplementary Fig. 6A–H ). Moreover, since the data do not fall on a line, an additional task might not be in trade-off. Metabolic efficiency While the performance frontier provides phenomenological insights into accession-specific trade-offs, it does not reveal whether and how the observed phenotypic performance relates to underlying cellular processes such as metabolism. In the following, we consider the metabolism of each accession as a production line that allocates the available resources, captured by metabolite and enzyme activity profiles, between two contending tasks: maximizing fresh weight and maximizing protein concentration. Although only a fraction of the metabolic phenotype can be measured, due to the high connectivity in metabolic networks [34] , the profiles carry information about other unmeasured traits [41] . Regression-based analyses have shown that metabolite and enzyme activity profiles provide an integrative metabolic phenotype that is predictive of biomass [33] , [34] , [42] , [43] , heterosis [44] , and, to a lesser extent, abiotic stress tolerance in plants [45] . In the following, we employ the Pareto efficiency principle for production systems [30] to test whether the trade-off between fresh weight and protein concentration is related to changes in resource availability and allocation in metabolism. Within this conceptual framework, an accession can be considered to be metabolically efficient if an attempt to further decrease any of its metabolic resources (inputs) or further increase any of the tasks (outputs) adversely affects other inputs or outputs, relative to all other considered accessions. Metabolically efficient accessions can be identified by solving a series of linear optimization problems integrating measurements of the inputs and outputs in the framework of data envelopment analysis (DEA). The metabolically efficient accessions define the efficiency frontier; it envelops the remaining accessions that are referred to as metabolically inefficient. As in the analysis based on the performance frontier, the identification of metabolically efficient accessions is contingent on the investigated tasks, accessions and conditions. In addition to discriminating metabolically efficient from inefficient accessions, this approach allows inefficient accessions to be ranked based on their distance from the efficiency frontier. Recent refinements of DEA based on the concept of super-efficiency [46] , [47] also make it possible to provide a ranking of the accessions that are deemed fully efficient. As a result, the metabolically efficient accessions receive a value of at least one, while the inefficient a positive value smaller than one. Metabolic profiling provides a high-dimensional metabolic phenotype. To determine the metabolic efficiency of accessions we used a method that couples principal component analysis (PCA) with DEA, referred to as PCA–DEA [48] , [49] . Using the principal components (PCs) that explain 70% of the variance in the condition-specific metabolic phenotypes as inputs and fresh weight and protein concentration as two contending outputs, we identified 15, 25 and 47 efficient accessions under OpN, LiN and LiC conditions, respectively ( Fig. 3 ). This indicates that many accessions are able to adjust their metabolism to different C and N supplies. The smallest number of metabolically efficient accessions was found in OpN. This might suggest that most of the Arabidopsis accessions are more adapted to limiting rather than near-optimal resources, or that other factors unrelated to the metabolic phenotype increase in importance when C and N are less limiting for growth. Figure 3: Venn diagram of the number of efficient accessions under the three conditions. The number of efficient accessions based on the results from PCA–DEA with 70% of variance explained for the two outputs, fresh weight (FW) and protein concentration under OpN (red), LiN (yellow) and LiC (blue) conditions as well as shared efficient accessions between different conditions is presented in white. The Kendall tau correlation coefficient is presented in black. Significant Kendall tau correlation ( P value <0.05, z A -statistic) is marked with a star. Full size image We next explored whether the growth condition influences metabolic efficiency of the accessions. To do this we determined the Kendall tau correlation, which takes values in the range between −1 and 1 and quantifies the correspondence between two rankings; in this case, the metabolic efficiencies of accessions in two growth conditions. This analysis yielded rather low but significant Kendall tau values in OpN versus LiN (0.20; P value=0.0043, z A -statistic) and OpN versus LiC (0.16; P value=0.0191, z A -statistic) comparisons and a very low and non-significant value in the LiN versus LiC (0.06; P value=0.3530, z A -statistic) comparison ( Fig. 3 ). This indicates that accession efficiency is condition-dependent. The especially low congruence between LiN and LiC is expected, as these are the most contrasting growth conditions. We asked which metabolic traits contribute most strongly to metabolic efficiency for fresh weight and for protein concentration. To this end, we determined the Kendall tau correlation between the ranking of accessions obtained with the full metabolic phenotype and the ranking obtained with a metabolic phenotype from which a given metabolic trait was excluded [50] : in this case, the lower the congruence, the higher the contribution of the omitted metabolic trait to accession efficiency in that condition. This was repeated for each metabolite, and for each condition and task ( Supplementary Fig. 7 ). The most strongly contributing metabolic traits are glucose, fructose and xylose under OpN; urea, chlorophyll b and glutamine oxoglutarate aminotransferase (GOGAT) under LiN, and threonine, sucrose and phospho enol pyruvate carboxylase (PEPCx) under LiC. These traits may be proxies that are closely linked to key metabolic traits that are not captured in our experimental analysis. Nevertheless, it is noteworthy that the most contributing metabolites in OpN include glucose and fructose, two important sugars that often accumulate when carbohydrates are high. In LiN they include urea and chlorophyll b, which are two key N-containing metabolites, and GOGAT, a key enzyme in N assimilation. In LiC they include sucrose, which is the transport sugar in plants, and PEPCx, which plays a key role in the synthesis of organic acids and amino acids. These findings demonstrate that not only the metabolic efficiencies of Arabidopsis accessions but also the metabolic traits that determine these efficiencies depend on the environmental condition. They also hint at a connection between metabolic plasticity and the robust trade-offs observed in the three conditions. Comparison across the three conditions revealed that while the majority of accessions were efficient in only one or two conditions, five accessions ( Bay-0 , Est-1 , Lan-0 , Lov5 and Wei1 ) were efficient under all three conditions. Three of these consistently metabolically efficient accessions ( Est-1 , Lov5 and Wei1 ) were located closest to the average performance frontier (distance to performance frontier <0.001) ( Fig. 2 ), highlighting them as showing a particularly strong trade-off in their response to the three environments, and one was fairly close to the average performance frontier ( Bay-0 ). Two ( Lov5 , Wei1 ) were the best average performers for fresh weight and protein concentration, respectively. The positions of these five consistently efficient accessions suggest that there may be a relationship between the performance frontier and the efficiency frontier. To address this issue, we tested the null hypothesis that the average fresh weight of the set of metabolically efficient accessions is not higher than the average fresh weight over the inefficient accessions. For the three growth conditions, the statistical test ( P value <0.05, t -distribution) was in favour of the alternative hypothesis, indicating that efficient accessions tend to have higher fresh weight ( Supplementary Fig. 8A–C ). This relationship does not hold for the protein concentration ( Supplementary Fig. 9A–C ), which is in line with the small overall negative correlation between fresh weight and protein concentration. These analyses led us to posit that accessions with a larger metabolic efficiency are closer to the performance frontier. To test this hypothesis, we determined the Kendall tau correlation between the distances of accessions from the performance frontier and their mean metabolic efficiencies in the three conditions. The negative correlation of −0.30 ( P value=0, z A -statistic, Supplementary Fig. 10 ) indicates that accessions with a stronger trade-off between fresh weight and protein concentration are also more efficient in using the metabolic phenotype towards achieving these two contending tasks. The finding that there is a statistically significant relation between the performance and efficiency frontiers supports the validity of our approach. It also points to metabolism playing an important role in the trade-off between fresh weight and protein concentration. We next investigated possible explanations for the observation that accessions with higher metabolic efficiency are closer to the performance frontier. We hypothesized that enhanced trade-offs and larger metabolic efficiency is associated with high metabolic plasticity. To explore this idea, we performed the following analysis for each accession: For each metabolic trait, we determined the log-fold change in each pair-wise comparison of the three conditions ( Supplementary Fig. 11A ) and then calculated the average log-fold change over the three pair-wise comparisons to provide a quantitative proxy for the accession-specific plasticity for that metabolic trait. The values for each metabolic trait were combined and plotted to provide an overview of the condition-dependent variation of each metabolic trait in a given accession ( Supplementary Fig. 11B ). This procedure was carried out for each of the analysed accessions ( Supplementary Fig. 11C ). The resulting distributions characterize the plasticity of the metabolic phenotype in an accession-specific manner. We investigated two properties of the distributions: skewness and 95th percentile. The skewness quantifies the extent to which the median of a distribution is shifted to one side of the mean: positive skewness is expected when majority of the metabolic traits show plasticity smaller than the mean ( Supplementary Fig. 12 ). The skewness was positive in all accessions, with an average skewness of 2.3365 (s.d. 0.4035) over all accessions ( Supplementary Table 5 ). Altogether, these results indicated that majority of metabolic traits show plasticity lower than the mean, and that this was the case for all accessions. This led us to focus on the metabolic traits that are in the right tail of the distributions, that is, those with plasticity greater than the mean. To do this, we employed the 95th percentile, the quantity below which 95% of the values in the distribution fall: the larger its value, the more extreme the plasticity of few metabolic traits. The average 95th percentile of the accessions was 2.7744 with a s.d. of 0.2796. This finding supports the earlier observation that majority of traits show a relatively small average log-fold change. We next tested whether the 95th percentiles of the distributions correlate with the distance of accessions to the performance frontier ( Supplementary Fig. 11D,E , Supplementary Table 5 ). The negative correlation (Kentall tau of −0.14, P value=0.0360, z A -statistic) indicated that accessions with a higher plasticity in a small number of metabolic traits are indeed closer to the performance frontier. Metabolic traits that showed average log-fold changes larger than the 95th percentile included are the following: spermidine, nitrate (NO 3 ), raffinose and dehydroascorbate in the majority of accessions (including the five consistently efficient across the three conditions) while arginine, glutamate, glutamine, glycine, isoleucine, proline-4-hydroxy and maltose were highly plastic in only few accessions ( Supplementary Table 5 ). Previous studies have implicated these metabolites as changing as a result of C or N limitation [51] , [52] . Altogether, these findings indicate that accessions that are more metabolically efficient exhibit more pronounced plasticity in a small number of metabolic traits, and are positioned closer to the performance frontier. Investigation of metabolic efficiencies also led to ask why the distribution of accessions around the performance frontier is highly unbalanced ( Fig. 2 ). One possibility is that many of the accessions are only adjusted to one condition in which they are metabolically efficient. However, this cannot be the full explanation because 34 accessions are metabolically inefficient in all three conditions ( Supplementary Table 6 ). A more likely explanation is that growth and survival of Arabidopsis requires the performance of further tasks that are not considered in our study, and that the importance of these unconsidered tasks varies, depending on the accession and environment. To test the hypothesis that other tasks may be in trade-off, we used scores that are publically available for 199 Arabidopsis accessions for sets of germination, defence-related, ionomics, developmental and flowering traits [53] . We investigated five scenarios with accessions that had full data sets for at least 50 traits ( Supplementary Fig. 13A–E ). In the first three scenarios, missing values were imputed for all traits (excluding germination) over all remaining accessions, and the criterion of triangulation was applied on all traits, defence and developmental, but only for the 41 accessions also present in our data set ( Supplementary Table 7 ). In the last two scenarios, the missing values were imputed only for the defence and developmental traits, and statistical tests were applied with all accessions and only the 41 accessions present also present in our data set. Interestingly, the criterion of triangularity was significant in the scenarios of defence and developmental traits for the 41 accessions with missing values imputed based on all or only defence and developments traits ( P values=0.0033 and 0, respectively, permutation test with 10,000 repetitions). Altogether these findings highlight two main aspects—first, the analysis in Shoval et al . [16] , like ours, is contingent on the data used and genotypes employed; second, some defence and developmental-related tasks might be in trade-off with increasing rosette sie and the protein concentration. However, this statement is not conclusive on the basis of the current study alone. To further investigate the latter claim, we determined the Kendall tau correlation between fresh weight for each growth condition, and the scores for the defence-related, ionomics, developmental and flowering traits investigated above. The hypothesis is that traits that are in trade-off with fresh weight will be negatively correlated to fresh weight. Validation of this hypothesis would provide further correlation-based support for the idea that other tasks, scored with the determined traits, are in trade-off with fresh weight or protein concentration, and may also be important for survival of the accessions. The strongest negative median correlation was observed between flowering traits and fresh weight, particularly under OpN and LiN ( Supplementary Fig. 14 , see Supplementary Tables 8-11 for individual traits). We repeated this procedure with protein concentration. For protein concentration, the strongest negative median correlation was observed for developmental traits, followed by defence-related and flowering phenotypes ( Supplementary Fig. 15 , see Supplementary Tables 12–15 for individual traits). It is noteworthy that the strongest negative correlations to metabolic efficiencies were also with flowering traits under OpN and LiN, followed by negative values of smaller magnitude for the developmental phenotype ( Fig. 4 , see Supplementary Tables 16–19 for individual traits). This indicates that under OpN and LiN, flowering traits may act as contending tasks with fresh weight and protein concentration among the accessions. Flowering traits are determined by a complex network that integrates many environmental and internal inputs [54] . Notably, the CONSTANS (CO)-FLOWERING LOCUS T(FT) photoperiod floral pathway operates in a 12-h photoperiod that was used in the OpN and LiN treatments, but not in the 8–h photoperiod that was used in the LiC growth condition. The relationship between metabolic efficiency and flowering phenotypes is in line with recent evidence for a connection between metabolism, via the sucrose signal metabolite trehalose 6-phosphate and the CO-FT photoperiod floral pathway [55] . This relationship is further supported by recently discovered links between metabolism and the transition to maturity, which is a prerequisite for flowering [55] , [56] , [57] . A link between metabolic efficiency and defence-related phenotypes may not be apparent in our analyses, due to either the experimental design or the possibility that defence response may be induced rather than constitutively related to metabolism. 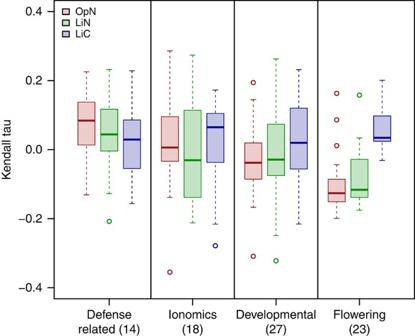Figure 4: Boxplots of Kendall tau coefficients from correlating the efficiencies with different phenotypes. The correlation between efficiencies under OpN (red), LiN (green) and LiC (blue) with defence-related, ionomics, developmental and flowering phenotypes, respectively, is presented in boxplots. The bottom and top of each box represent the first and third quartiles of the distribution of the Kendall correlation coefficient, respectively. The horizontal line inside each box is the median (second quartile). The whiskers range between ±1.58 IQRn−1/2, where IQR is the interquartile range andnis the number of points in the distributions. Data points outside this range are considered as outliers, indicated as circles. The number of accessions considered in each phenotype is presented in parenthesis. Figure 4: Boxplots of Kendall tau coefficients from correlating the efficiencies with different phenotypes. The correlation between efficiencies under OpN (red), LiN (green) and LiC (blue) with defence-related, ionomics, developmental and flowering phenotypes, respectively, is presented in boxplots. The bottom and top of each box represent the first and third quartiles of the distribution of the Kendall correlation coefficient, respectively. The horizontal line inside each box is the median (second quartile). The whiskers range between ±1.58 IQR n −1/2 , where IQR is the interquartile range and n is the number of points in the distributions. Data points outside this range are considered as outliers, indicated as circles. The number of accessions considered in each phenotype is presented in parenthesis. Full size image Natural variation in A. thaliana is a useful resource to identify and investigate mechanisms that underlie trade-offs between tasks in different environments. However, it is a challenge to interpret the multidimensional data sets that are generated by studies of trade-offs. While correlation-driven methods can be used to identify trade-offs, they do not allow the comparison of genotype-specific trade-offs in and across multiple environments. Here we use the Pareto frontier concept to uncover accession-specific differences in performance, and rank accessions for metabolic efficiency, both in and between environmental conditions. We demonstrate that some accessions are efficient across a range of conditions. We also show that metabolically efficient accessions are close to the average performance frontier in a range of growth conditions, demonstrating that there is considerable agreement between these two approaches. Further, accessions that lie closer to the average performance frontier show a higher metabolic plasticity for a small subset of metabolic traits, providing first insights into which features of metabolism contribute to phenotypic plasticity. Altogether, our findings indicate a relation between plasticity of metabolic phenotypes, metabolic efficiency and contending growth-related tasks. This approach can be readily extended to investigate a wider range of tasks, environmental conditions and molecular phenotypes in different species. Description of the selection of used accessions and growth conditions as well as metabolite and enzyme assays can be found in Supplementary Methods . Genetic distance The genetic distances between accessions are determined based on the most comprehensive information existing about polymorphisms (200,155 SNPs) [58] . This is available for 73 of the 97 investigated accessions. The resulting distance matrix was used to build a tree by using a neighbor-joining algorithm [59] . Although the main branches partially separate the accessions according to the geographic origin (for example, Northern, Western, Eastern and Southern Europe), there is still some admixture. A similar grouping pattern to ours was reported in a study that used a comparable number of markers and accessions [53] . Data envelopment analysis DEA is a computational approach, based on linear programming (LP), which aims at determining the relative efficiency of entities, so-called decision-making units (DMUs), specified with their respective inputs and outputs. In our framework, the DMUs correspond to the different Arabidopsis accessions. In contrast to other approaches for analysis of multidimensional data, allowing only pair-wise combination of biochemical system levels (for example, metabolites and transcripts, or proteins and metabolites), DEA is applicable across data from multiple levels of biological organization. With the help of DEA, one can readily identify the best-performing accession by providing a ranking based on the relative efficiency. Here we extend this approach to determine the reasons (represented by particular metabolic traits) responsible for the performance of a particular accession. As opposed to other approaches for analysis of multivariate data, DEA considers all input and all output levels simultaneously. To quantitatively combine the multiple inputs and multiple outputs, DEA computes the relative efficiency of each individual accession with respect to all other accessions by employing the weighted averages, so that: While this leads to respective aggregations of inputs and outputs, we point out that, unlike in other statistical techniques for multivariate data analysis, the aggregations in DEA differ between accessions. Consider a set of s accessions with each accession α , 1≤ α ≤ s , with m inputs , 1≤ i ≤ m , generating n outputs , 1≤ j ≤ n . The efficiency of a particular accession a is then given by the solution of a fractional programme, originally proposed by [60] : where v i and μ j correspond to the weights associated with the input i and the output j , respectively. We point out that this model, maximizing the linear combination of outputs without requiring more of any of the observed inputs, is referred to as the input-oriented model. Clearly, the reciprocal of the ratio of inputs to outputs results in another type of model, named output-oriented, which minimizes the inputs while producing at least the given output levels [30] . We note that the qualitative findings from the input- and output-oriented models, with respect to the ranking of accessions based on the relative efficiencies, are equivalent. With the help of the theory of fractional programming [61] , the fractional programme in Equation (2) can be formulated as a LP problem by constraining the denominator of the objective function to one and only minimizing the numerator. Depending on the scale assumptions in calculating the relative efficiencies, there are two basic DEA models, the CCR ( C harnes, C ooper and R hodes) model [60] and its extension the BCC ( B anker, C harnes and C ooper) model [62] . The former formalizes the concept of constant returns to scale, whereby the output changes by the same proportion as the input. On the other hand, the latter captures the concept of variable returns to scale (VRS), comprising the three variants, namely increasing-, decreasing- and constant returns to scale. Clearly, any CCR-efficient accession is also BCC-efficient. As a result, in the following, we focus on the more general BCC model to consider also the effects of increasing- and decreasing returns to scale. The LP formulation for the BCC model is defined as follows: By the duality theorem, this problem is equivalent to the following LP: where s i and s j are the slacks of the input i and the output j , respectively, used to convert the inequalities into equivalent equations and Θ a gives the efficiency score for accession a . The vector λ represents the weights of the accessions resulting from the LP given in Equation (4). By the strong duality theorem, the optimal value of the dual problem, given in Equation (4), equals the optimal value of the primal problem in Equation (3). The number of constraints for the primal programme depends on the number of accessions, while that of the dual programme depends on the number of inputs and outputs. An accession a is considered (fully) BCC-efficient in the VRS sense if there exists a solution to Equation (4) such that the following two conditions are satisfied: 1 Θ a =1. 2 All slacks s i , 1≤ i ≤ m , and s j , 1≤ j ≤ n , are zero. These two conditions define the so-called Pareto–Koopmans efficiency, whereby an accession is fully efficient when an attempt to improve on any of its inputs or outputs will adversely affect some other inputs or outputs. The efficient accessions define the Pareto efficiency frontier [30] . Combination of PCA and DEA If the number of analysed accessions, s , is less than the total number of inputs and outputs, m + n , a large number of accessions may be predicted to be efficient (depending on the structure of the data set). To resolve this issue, arising due to the multidimensionality of the data, the number of constraints imposed in the formulation of DEA in Equation (3) needs to be reduced. Consequently, DEA has been combined with PCA to reduce the dimension of inputs and outputs while minimizing the loss of information [48] . PCA is a linear algebra technique that can be used to represent a set of possibly correlated variables into a set of uncorrelated variables called PCs. Each PC is represented as a linear combination of the original variables. The coefficients in the linear combination are given by the eigenvectors from the eigenvalue decomposition of the covariance matrix for the analysed set of variables. The PCs are usually ordered by the percentage of the accounted variance, starting with the component of the largest variance. It should be noted that the number of PCs is less than or equal to the number of original variables [63] . The variance ζ k , (1≤ k ≤ K ) explained by the k th PC is calculated as: where K is the number of original variables and φ l , (1≤1≤ K ) is the l th largest eigenvalue of the covariance matrix for the K variables. The number of PCs used in analyses depends on the percentage of variance to be explained for a particular purpose. Indeed, considering all PCs amounts to using the original data set. Formulation of PCA–DEA The usage of PCs instead of the original data induces a transformation of the DEA model. Therefore, the inputs X and the outputs Y are transformed through PCA. Let and denote the matrices containing the coefficients of the linear combinations rendering the PCs of the input and output data, respectively. The size of this matrix is reduced to the number of PCs that explain a pre-specified percentage of the variance in the original data. Then, and are the k PCs, that is, linear combinations, of the variables in the data sets X and Y . Furthermore, the number of columns in X k and Y k correspond to the number k of PCs used to represent the input and output data. Consequently, the general BCC model from Equation (3) for accession a can be transformed as follows: where U 0 and V 0 represent the vectors of weights for the inputs and outputs, respectively, used with their original values, while U k and V k denote the coefficients of the PCs used for the input and output data. Since , where V k represents a row vector of dual variables, the weights of the original input X can be expressed as . We note that the same holds for the output. Furthermore, the corresponding dual programme can be rewritten as follows: The problem in Equation (7) is referred to as the envelopment problem. Like the primal programme given in Equation (6), it provides weights for each accession, indicating those accessions of highest influence to the efficiency of the accession a for which the efficiency is calculated. Since the number of outputs is really small in the considered data set PCA is only applied on the inputs. Therefore, all constraints containing X and as well as Y k and are not included in the linear programs. As suggested by Adler et al . [64] all the values are divided by the corresponding s.d. The correlation matrix of standardized inputs and PCs are calculated and finally the linear programs are used to derive efficiency scores. Ranking of efficient accessions The general results of DEA and also PCA–DEA group the accessions into two sets, those that are efficient and therefore define the Pareto efficiency frontier and those that are inefficient. In order to obtain a complete ranking of all accessions, another approach or modification is required. Many mathematical and statistical techniques have been developed to rank both efficient as well as inefficient DMUs in our case accessions. Adler et al . [65] provide an overview about the general ranking methods applied in economics. Among others one approach to the ranking problem is that provided by the super-efficiency model, first published by Andersen and Petersen [46] . The super-efficiency model involves executing the standard DEA model (in our case VRS PCA–DEA), but under the assumption that the accession, a , being currently evaluated is excluded from the reference set. In the input-oriented case the model provides a measure of the proportional increase in the inputs for an accession that could take place without destroying the ‘efficient’ status of that accession relative to the frontier created by the remaining accessions. The unit obtains in that case an efficiency score above one. The methodology enables an extreme efficient unit f to achieve an efficiency score greater than one by removing the f th constraint in the primal formulation. A problem of the calculation of super-efficiency is that it is well known that under certain conditions, the super efficiency DEA model may not have feasible solutions for efficient accessions. As shown for instance by Seiford and Zhu [66] as well Dulá and Hickman [67] , infeasibility must occur in the case of the VRS super-efficiency model. The model of Lovell and Rouse [47] identify and provide a feasible solution for all super-efficient units that are infeasible in the conventional VRS super-efficiency model. This modified DEA scales up the inputs (down the outputs) of the accession under evaluation. The super-efficiency scores for all efficient accession without feasible solutions are then equal to the user-defined scaling factor β . The modified super-efficiency model is defined as follows: Note that the scalar β >1 must be sufficiently large to make it inefficient to ensure that e a <1. This is not guaranteed if the accession e a <1 is extreme-efficient, which would lead to infeasibility for the general super-efficiency model and an efficiency score of 1, e a =1, for the modified super-efficiency model of Lovell and Rouse [47] . We further extend this modified super-efficiency model to use it also to rank the efficient accessions of the PCA–DEA approach, which has to deal in general with the same problems as the conventional DEA. Then, for ranking the accessions of the input-oriented VRS PCA–DEA we use the model as follows: Statistical analysis The Kendall rank correlation coefficient, denoted by τ , evaluates the degree of similarity between two sets of ranks over the same set of objects [68] . It can be determined by the following expression: where a pair of ranked sets ( x i , y i ) and ( x j , y j ) (on the same set of objects) is concordant if the order of both objects agree, that is, if both x i > x j and y i > y j or x i < x j and y i < y j . In contrast, a pair is discordant, if x i < x j and y i > y j or if x i > x j and y i < y j . If x i = x j or y i = y j , the pair is neither concordant nor discordant. Larger (positive) values of τ indicate a greater agreement between the two sets, while smaller (negative) values imply disagreement. We use the Kendall rank coefficient in order to capture the effect of a particular input on the resulting ranking of the accessions based on PCA–DEA. To this end, the influence of an input parameter t on the relative efficiency of a given accession under a condition c is determined by excluding t from the inputs and applying PCA–DEA to obtain the efficiencies under condition c . We then use Kendall’s τ to qualitatively discriminate between different inputs (that is, metabolic traits) with respect to their correspondence to the obtained efficiencies, resulting in: where e c are the efficiencies including all inputs. Investigation of metabolic plasticity For the 48 metabolite and eight enzyme activity profiles the absolute values of log-fold changes, FC between a pair of conditions c i and c j are calculated by: The average FC over the three pairs of conditions (that is, OpN/LiC, OpN/LiN and LiN/LiC) is calculated as an indicator for the plasticity of each metabolic trait in the investigated conditions. For every accession the distribution of average absolute values of log-fold changes over all metabolic traits is then determined. Furthermore, the skewness of the resulting distributions is calculated as follows: where n is the number of observations included in the distribution and is the mean of observations, here, of average absolute values of FC for 56 metabolic traits. A negative value of the skewness denotes a longer left tail and a larger median of the distribution, whereas positive values indicate a longer right tail and a smaller median, respectively. In addition, the 95th percentile, capturing the distribution of values in the right tail of each distribution, is used to quantify the overall plasticity of metabolic traits showing large plasticity in the three conditions. Investigation of the criterion of triangularity We followed the approach of Shoval et al . [16] by making use of the Pareto front software. To this end, we investigated the findings from five scenarios: The data set of Atwell et al . [53] includes 199 accessions and five types of traits: defence-related, ionomics, developmental, flowering and germination traits. From this list, we excluded the categorical traits with binary values as well as the germination traits (as they are expected to have small effect on the later vegetative plant growth). We note that 41 of these accessions are also present in the set of genotypes that we analysed in our study ( Supplementary Table 7 ). Scenario I: we removed 29 out of 199 accessions that did not contain data about at least 50 traits; the missing values for the remaining accessions were imputed for all traits by using the most recent robust imputation method suitable for mixed data types (that is, categorical and continuous) based on random forests via the missForest R package [69] ; Scenario II: we removed 29 out of 199 accessions that did not contain data about at least 50 traits; the missing values for the remaining accessions were imputed for all traits by using random forests imputation method; finally, only defence traits and developmental traits were used; Scenario III: like Scenario II but only for the 41 accession in the overlap between our set of genotypes and the population used in Atwell et al . [53] ; Scenario IV: we removed 29 out of 199 accessions that did not contain data about at least 50 traits; the missing values for the remaining accessions were imputed for only defence traits and developmental traits by using random forests imputation method via the missForest R package [69] ; and Scenario V: like Scenario IV but only for the 41 accession in the overlap between our set of genotypes and the population used in Atwell et al . [53] . These five scenarios were necessary to control and investigate the effects of missing values and the way in which they were imputed. We note that the germination traits were removed from the analysis in all five scenarios to also facilitate the comparison of findings and the application of PCA (requiring more accessions than traits in Scenarios III and V). Implementation All mathematical programming approaches are implemented in MATLAB 7.11.0. We use CPLEX v12.2 to solve the considered LP problems. Statistical analysis was conducted in the R 2.15.2 environment for statistical computing. How to cite this article: Kleessen, S. et al . Metabolic efficiency underpins performance trade-offs in growth of Arabidopsis thaliana . Nat. Commun. 5:3537 doi: 10.1038/ncomms4537 (2014).